Next-generation muscle-directed gene therapy by in silico vector design There is an urgent need to develop the next-generation vectors for gene therapy of muscle disorders, given the relatively modest advances in clinical trials. These vectors should express substantially higher levels of the therapeutic transgene, enabling the use of lower and safer vector doses. In the current study, we identify potent muscle-specific transcriptional cis -regulatory modules ( CRMs ), containing clusters of transcription factor binding sites, using a genome-wide data-mining strategy. These novel muscle-specific CRMs result in a substantial increase in muscle-specific gene transcription (up to 400-fold) when delivered using adeno-associated viral vectors in mice. Significantly higher and sustained human micro-dystrophin and follistatin expression levels are attained than when conventional promoters are used. This results in robust phenotypic correction in dystrophic mice, without triggering apoptosis or evoking an immune response. This multidisciplinary approach has potentially broad implications for augmenting the efficacy and safety of muscle-directed gene therapy. Hereditary muscle disorders are characterized by significant morbidity and mortality due to skeletal muscle and cardiac dysfunction [1] . Most of these diseases lack effective treatment, which underscores their unmet medical need. In view of recent clinical successes [2] , [3] , [4] , [5] , gene therapy offers promising therapeutic perspectives for many genetic diseases, including muscle disorders. Most importantly, muscle-directed gene therapy constitutes the basis of the first regulatory approved gene therapy product [6] , [7] , [8] , [9] . Most common hereditary muscle disorders are caused by single gene defects. In particular, Duchenne muscular dystrophy (DMD) affects 1 in 3500 live newborn males and is caused by mutations in the dystrophin ( DYS ) gene [10] . Patients typically die at an early age from cardiopulmonary failure after progressive muscle deterioration [11] . Long-term expression and therapeutic effects have been reported after gene therapy using adeno-associated viral vectors (AAVs) in animal models [12] , [13] , [14] , [15] . Typically, for gene therapy of DMD, truncated versions of the dystrophin gene are used (i.e., micro-dystrophin) [16] , [17] that can readily be accommodated into these AAV vectors. In addition to correcting muscle diseases per se, the muscle is also an attractive target for delivery of secreted proteins into the circulation after gene therapy given its secretory capacity [18] , [19] . Despite its promise, it has been particularly challenging to achieve robust and widespread expression of a given therapeutic gene in the skeletal muscle [18] , [20] , [21] , [22] . For instance, clinical trials for DMD establish proof of concept that targeting the muscle by gene therapy is feasible, though the overall therapeutic benefits were limited [20] , [23] . Moreover, muscle-directed oligonucleotide-mediated exon-skipping strategies did not yet yield the expected outcome in pivotal trials in patients suffering from DMD [24] , [25] , despite increased dystrophin-expression [26] , [27] . Though increasing the vector doses may result in more efficient gene transfer, this concomitantly increases the risk of triggering inadvertent immune reactions [28] , [29] . Hence, to overcome these limitations, it is mandatory to develop more potent gene therapy vectors containing novel promoters that outperform conventional ones [22] , [30] , [31] and that consequently allow for high and widespread muscle-specific expression at lower and safer vector doses. In the current study, we use genome-wide data-mining to identify robust transcriptional cis -regulatory modules ( CRMs ) that are effective in boosting transcriptional targeting up to 400-fold in skeletal muscle. This multidisciplinary approach provides new insights into regulatory motifs and their relative strength in conferring muscle-specific transcriptional control. These novel muscle CRMs increase expression of micro-dystrophin (MD1) [16] , [17] and follistatin (FST344), a known myostatin inhibitor [32] , after gene therapy with serotype 9 adeno-associated viral vectors (AAV9) [33] , [34] . This results in sustained phenotypic correction in dystrophic mice without any discernable immune complications. Computational identification of Sk-CRM To design robust muscle-specific gene therapy vectors, we relied on a multistep computational approach (Fig. 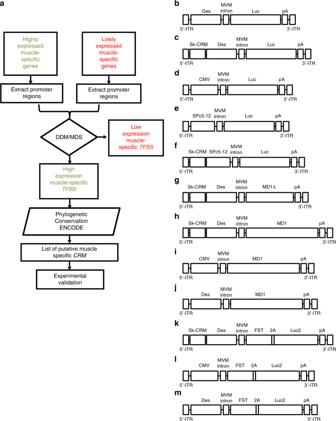Fig. 1 Flow diagram for the identification of muscle-specificcis-regulatory modules (CRMs) and AAV constructs for in vivo validation.aA computational approach was used to identify theSk-CRMsinvolving the following five steps: (1) identification of tissue-specific genes that are highly and lowly expressed based on statistical analysis of micro-array expression data of normal human tissues; (2) extraction of the corresponding promoter sequences from publicly available databases; (3) identification of theCRMsand the transcription factor binding sites (TFBS) they contain using a differential distance matrix (DDM)-multidimensional scaling (MDS) approach; (4) search for evolutionary conserved clusters ofTFBS(i.e.,CRM) of the highly expressed genes (5) ENCODE filtering. The identifiedSk-CRMswere subsequently included in an expression construct and validated in vivo by testing whether they increased promoter activity.b–mSchematic representation of all the different AAV vectors encoding either the reporter or therapeutic genes. The different expression cassettes were packaged in an adeno-associated virus vector flanked by inverted terminal repeats (ITR) from AAV serotype 2 (AAV2) and produced with an AAV serotype 9 (AAV9) capsid. The expression cassette further comprises the Minute Virus of Mouse (MVM) intron and a Simian virus 40 (SV40) polyadenylation signal (pA).bThe scAAV-Des-Luc vector is a self-complementary AAV vector (scAAV) containing the luciferase (Luc)gene driven from the desmin (Des) promoter without the CRM used as a controlcthe scAAV-Sk-CRM-Des-Luc vectors contain theSk-CRM 1-7cloned upstream theDespromoter.dThe scAAV-CMV-Luc vector uses theCMVpromoter to drive theLucgene.eThe scAAV-SPc5-12-Luc vector has the same vector configuration as inbwhere theDespromoter was replaced by theSPc5-12promoter.fThe scAAV-Sk-CRM4-SPc5-12-Luc vector contains theSk-CRM4element cloned upstream of theSPc5-12promoter driving the expression of theLucgene. The single-stranded AAV (ssAAV) vectors were used to deliver therapeutic genesg–jmicro-dystrophin (MD1Δ orMD1) andk–mthe follistatin (FST344), respectively, withSkCRM4/Deschimeric promoter or CMV andDesconventional promoters. The cognate FST protein is encoded by aFST-2A-Lucpolycistronic transcript 1a ) that allowed us to identify novel evolutionary conserved skeletal muscle-specific cis -regulatory modules (designated as Sk-CRMs ) associated with genes that are highly expressed in the skeletal muscle (Table 1 and Supplementary Table 1 ). Using this computational approach, we have identified seven different Sk-CRMs based on human sequences ranging from sizes 344 bp to 519 bp (Table 1 , Supplementary Table 1 , and Supplementary Fig. 1 ). These Sk-CRMs comprised binding sites for seven different transcription factors (TFs) including E2A, CEBP, LRF, MyoD, SREBP, Tal1, PPAR (Table 1 ; Supplementary Fig. 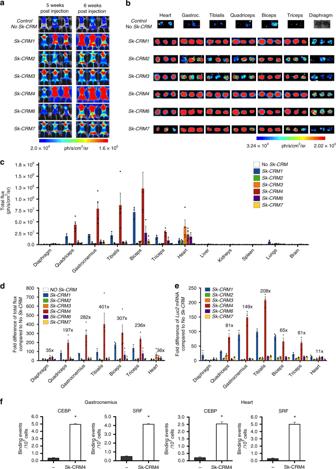Fig. 2 Screening and validation of novel hyperactiveSk-CRMs. CB17/IcrTac/Prkdcscidmice were intravenously injected with 5 × 109vg per neonatal mouse.aIn vivo whole-body bioluminescence imaging of mice injected intravenously with scAAV9-Des-Luc2 (control, noSk-CRM), scAAV9-Sk-CRM1-Des-Luc (Sk-CRM1), scAAV9-Sk-CRM2-Des-Luc (Sk-CRM2), scAAV9-Sk-CRM3-Des-Luc (Sk-CRM3), scAAV9-Sk-CRM4-Des-Luc (Sk-CRM4), scAAV9-Sk-CRM6-Des-Luc (Sk-CRM6), or scAAV9-Sk-CRM7-Des-Luc (Sk-CRM7) vector were shown based on a color scale from 2.0e + 04 (blue) ph/s/cm2/sr to 1.59e + 06 (red) ph/s/cm2/sr at week 5 and 6 post vector injection. Photon emission was measured dynamically during 7 min in a supine position.bEx vivo bioluminescence imaging of individual organs harvested at week 7 post vector injection was represented on a color scale with luciferase intensities ranging from 3.23e + 04 (blue) ph/s/cm2/sr to 2.05e + 05 (red) ph/s/cm2/sr. The bioluminescence signal was quantified for 5 min.cA hand-drawn region of interest (ROI) was used for every individual tissue. Luciferase expression from the individual muscles was measured as total flux, expressed in photons/sec/cm2/sr.dFold-difference of the total flux measured from the different muscles upon ex vivo bioluminescence imaging with respect to the control (construct withoutSk-CRM).eFold-difference inLucmRNA expression levels from the different muscles, measured by qRT-PCR from total RNA extracted from biopsies of the indicated tissues. Results were presented as mean ± standard error of the mean, fold-difference inLucmRNA expression with respect to the control (construct withoutSk-CRM).fChromatin immune-precipitation (ChIP) assay for the heart and gastrocnemius muscle of mice injected with scAAV9-Sk-CRM4-Des-Luc (5 × 109vg/mouse). Antibodies specific for CEBP and SRF and PCR primers specific for the correspondingTFBSwere used. PCR primers were designed to amplify a region corresponding toSk-CRM4that binds CEBP and SRF and an untranscribed region on chromosome 17 was used as a negative control. Binding events for 103cells were determined for each of the corresponding primer pairs. The black bars represent the negative control and the white bars correspond toSk-CRM4; heart (left panel), gastrocnemius (right panel). Significant differences compared to the negative control were indicated (t-test, *p≤ 0.05, mean + s.e.m.;n= 2–4) 1 , and Supplementary Table 2 ). The Sk-CRM elements (i.e., Sk-CRM1 to Sk-CRM7 ) corresponded to transcription factor binding site ( TFBS ) clusters in the promoters or introns of the following muscle-specific genes: ATP2A1 (Sk-CRM1), TNNI1 (Sk-CRM2, Sk-CRM3), MYLPF (Sk-CRM4); MYH1 (Sk-CRM5), TPM3 (Sk-CRM6), ANKRD2 (Sk-CRM7) (Table 1 , Supplementary Table 1 , and Supplementary Fig. 1 ). Several Sk-CRMs contain identical TFBS but each Sk-CRM is unique with respect to the specific TFBS arrangement. These distinct Sk-CRMs , therefore, contained a molecular signature that is characteristic of genes that are highly expressed in the muscle. The selected Sk-CRMs were relatively conserved in evolution (Supplementary Fig. 1 ), suggesting strong selective pressure to maintain these particular TFBS combinations to enable high muscle-specific expression. The use of these evolutionary conserved human Sk-CRMs increased the likelihood that their potency and specificity is preserved following clinical translation. Fig. 1 Flow diagram for the identification of muscle-specific cis -regulatory modules ( CRMs ) and AAV constructs for in vivo validation. a A computational approach was used to identify the Sk-CRMs involving the following five steps: (1) identification of tissue-specific genes that are highly and lowly expressed based on statistical analysis of micro-array expression data of normal human tissues; (2) extraction of the corresponding promoter sequences from publicly available databases; (3) identification of the CRMs and the transcription factor binding sites ( TFBS ) they contain using a differential distance matrix (DDM)-multidimensional scaling (MDS) approach; (4) search for evolutionary conserved clusters of TFBS (i.e., CRM ) of the highly expressed genes (5) ENCODE filtering. The identified Sk-CRMs were subsequently included in an expression construct and validated in vivo by testing whether they increased promoter activity. b – m Schematic representation of all the different AAV vectors encoding either the reporter or therapeutic genes. The different expression cassettes were packaged in an adeno-associated virus vector flanked by inverted terminal repeats (ITR) from AAV serotype 2 (AAV2) and produced with an AAV serotype 9 (AAV9) capsid. The expression cassette further comprises the Minute Virus of Mouse (MVM) intron and a Simian virus 40 (SV40) polyadenylation signal ( pA ). b The scAAV-Des-Luc vector is a self-complementary AAV vector (scAAV) containing the luciferase ( Luc) gene driven from the desmin ( Des ) promoter without the CRM used as a control c the scAAV-Sk-CRM-Des-Luc vectors contain the Sk-CRM 1-7 cloned upstream the Des promoter. d The scAAV-CMV-Luc vector uses the CMV promoter to drive the Luc gene. e The scAAV-SPc5-12-Luc vector has the same vector configuration as in b where the Des promoter was replaced by the SPc5-12 promoter. f The scAAV-Sk-CRM4-SPc5-12-Luc vector contains the Sk-CRM4 element cloned upstream of the SPc5-12 promoter driving the expression of the Luc gene. The single-stranded AAV (ssAAV) vectors were used to deliver therapeutic genes g – j micro-dystrophin ( MD1 Δ or MD1 ) and k – m the follistatin ( FST344 ), respectively, with SkCRM4/Des chimeric promoter or CMV and Des conventional promoters. The cognate FST protein is encoded by a FST-2A-Luc polycistronic transcript Full size image Table 1 Sequence and details of the Sk-CRMs Full size table In vivo identification of robust muscle-specific Sk-CRM An in vivo screening of these Sk-CRMs was subsequently performed to identify the most robust elements. To achieve this, we cloned the different Sk-CRMs upstream of a desmin ( Des ) promoter (Fig. 1b ) that drove the expression of a luciferase ( Luc ) reporter gene. The Des promoter was chosen since it is known to confer relatively high levels of skeletal muscle and heart-specific transgene expression [35] . The constructs were packaged using AAV serotype 9 (AAV9) to maximize skeletal muscle and cardiac-specific gene transfer [36] , [37] , [38] . The scAAV9-Sk-CRM-Des-Luc vectors containing either Sk-CRM1, Sk-CRM2, Sk-CRM3, Sk-CRM4, Sk-CRM6 , or Sk-CRM7 (Fig. 1c ) were then intravenously injected at a dose of 5 × 10 9 vg/mouse into neonatal CB17/IcrTac/Prkdc scid mice. Bioluminescence imaging revealed that 6 out of 6 (100%) (Fig. 2a–c ) different Sk-CRMs that were tested in vivo significantly augmented expression of the luciferase reporter gene from the Des promoter in distinct skeletal muscle groups but not in other organs. Most importantly, the Sk-CRM4 element resulted in an unprecedented and significant 200 to 400-fold increase ( t -test; p < 0.05) in luciferase expression (based on total photon flux) from the Des promoter in different muscle groups (i.e., gastrocnemius, tibialis, quadriceps, biceps, and triceps) (Fig. 2d ), compared to controls without Sk-CRM4 . This was consistent with a significant ( t -test; p < 0.01) 60 to 200-fold increase in Luc mRNA expression in these different muscle groups when the Sk-CRM4 was used in combination with the Des promoter (Fig. 2e ). Linear regression analysis confirmed a strong correlation between the luciferase activity and the Luc mRNA levels in the different muscle groups (correlation coefficient R 2 = 0.8). Interestingly, the Sk-CRM4 element also increased luciferase expression in the diaphragm (i.e., 35-fold) (Fig. 2b–d ) but to a lesser extent than in the other skeletal muscles. This difference likely reflects the lower intrinsic activity of the Des promoter in the diaphragm (Fig. 2b ). Alternatively, the reduced transduction efficiency with AAV9 in diaphragm compared to most of the other muscle groups may also have contributed to the difference in luciferase expression (Supplementary Fig. 2 ). Moreover, the selected Sk-CRMs also significantly increased expression in the heart, reflecting the tropism of AAV9 and the specificity of the Des promoter (Fig. 2b, c ). In particular, the most robust and significant ( t -test; p < 0.05) increase in cardiac expression was achieved with the Sk-CRM4 (i.e., 36-fold) or Sk-CRM3 elements (i.e., 65-fold) (Fig. 2d ). Fig. 2 Screening and validation of novel hyperactive Sk-CRMs . CB17/IcrTac/Prkdc scid mice were intravenously injected with 5 × 10 9 vg per neonatal mouse. a In vivo whole-body bioluminescence imaging of mice injected intravenously with scAAV9-Des-Luc2 (control, no Sk-CRM ), scAAV9-Sk-CRM1-Des-Luc ( Sk-CRM1 ), scAAV9-Sk-CRM2-Des-Luc ( Sk-CRM2 ), scAAV9-Sk-CRM3-Des-Luc ( Sk-CRM3 ), scAAV9-Sk-CRM4-Des-Luc ( Sk-CRM4 ), scAAV9-Sk-CRM6-Des-Luc ( Sk-CRM6 ), or scAAV9-Sk-CRM7-Des-Luc ( Sk-CRM7 ) vector were shown based on a color scale from 2.0e + 04 (blue) ph/s/cm 2 /sr to 1.59e + 06 (red) ph/s/cm 2 /sr at week 5 and 6 post vector injection. Photon emission was measured dynamically during 7 min in a supine position. b Ex vivo bioluminescence imaging of individual organs harvested at week 7 post vector injection was represented on a color scale with luciferase intensities ranging from 3.23e + 04 (blue) ph/s/cm 2 /sr to 2.05e + 05 (red) ph/s/cm 2 /sr. The bioluminescence signal was quantified for 5 min. c A hand-drawn region of interest (ROI) was used for every individual tissue. Luciferase expression from the individual muscles was measured as total flux, expressed in photons/sec/cm 2 /sr. d Fold-difference of the total flux measured from the different muscles upon ex vivo bioluminescence imaging with respect to the control (construct without Sk-CRM ). e Fold-difference in Luc mRNA expression levels from the different muscles, measured by qRT-PCR from total RNA extracted from biopsies of the indicated tissues. Results were presented as mean ± standard error of the mean, fold-difference in Luc mRNA expression with respect to the control (construct without Sk-CRM ). f Chromatin immune-precipitation (ChIP) assay for the heart and gastrocnemius muscle of mice injected with scAAV9-Sk-CRM4-Des-Luc (5 × 10 9 vg/mouse). Antibodies specific for CEBP and SRF and PCR primers specific for the corresponding TFBS were used. PCR primers were designed to amplify a region corresponding to Sk-CRM4 that binds CEBP and SRF and an untranscribed region on chromosome 17 was used as a negative control. Binding events for 10 3 cells were determined for each of the corresponding primer pairs. The black bars represent the negative control and the white bars correspond to Sk-CRM4 ; heart (left panel), gastrocnemius (right panel). Significant differences compared to the negative control were indicated ( t -test, * p ≤ 0.05, mean + s.e.m. ; n = 2–4) Full size image Despite the relatively broad tissue-tropism of AAV9 (Supplementary Fig. 2 ), luciferase reporter gene expression was mainly restricted to skeletal muscle and heart. In particular, liver, kidney, spleen, and the brain showed no or only limited luciferase expression with any of the Sk-CRMs (Fig. 2c and Supplementary Fig. 3 ). Nevertheless, low-level expression was apparent in the lung (Supplementary Fig. 3 ), albeit substantially less compared to that in skeletal muscle or heart (Fig. 2c ), particularly when the most robust Sk-CRM4 was employed. The computational algorithm predicted that Sk-CRM4 contained clusters of TFBS , including CEBP and SRF (Table 1 , Supplementary Tables 1 and 2 , and Supplementary Fig. 1 ). We, therefore, experimentally confirmed the binding of CEBP and SRF, on the most potent Sk-CRM4 element by chromatin immunoprecipitation (ChIP) using gastrocnemius muscle and heart from mice that were injected with the scAAV9-Sk-CRM4-Des-Luc vector. In particular, the ChIP assay revealed a significant 23-fold enrichment in the case of both CEBP and SRF on the Sk-CRM4 element over the negative control for the gastrocnemius muscle. Similarly, a specific 12-fold enrichment in case of CEBP and a 26-fold enrichment for SRF on the Sk-CRM4 element over the negative control were apparent in the heart (Fig. 2f ). Taking into account that the computational motif search tool estimates the overall probability of a TF binding to a given promoter region, these ChIP assay results suggest binding of the respective TFs on a promoter region of the MYLPF gene, that encompasses the corresponding TFBS elements. Hence, these ChIP assay results suggest that TF binding on the corresponding TFBS elements likely contributed to the increased transcriptional activity, which in turn resulted in higher protein expression levels. In vivo validation of Sk-CRM4 fragments Subsequently, we assessed whether smaller fragments of the computationally defined Sk-CRM4 element, were capable of producing an effect similar to what could be achieved with the full-length Sk-CRM4 . Moreover, since the initial screening was conducted in neonates (Fig. 2 ), it was important to also confirm the Sk-CRM4 effect in adult mice (Fig. 3 ). These Sk-CRM4 fragments (designated as Sk-CRM4 a , Sk-CRM4 b , Sk-CRM4 c , Sk-CRM4 d , and Sk-CRM4 e ) were identified by selecting out smaller fragments within the full-length Sk-CRM4 containing dense clusters of TFBS (Table 1 , Supplementary Fig. 1 , and Supplementary Table 1 ). The scAAV9-Sk-CRM-Des-Luc vectors (containing either the full-length Sk-CRM4 or its Sk-CRM4 a , Sk-CRM4 b , Sk-CRM4 c , Sk-CRM4 d , and and Sk-CRM4 e fragments) were then intravenously injected at a dose of 10 10 vg/mouse into adult CB17/IcrTac/Prkdc scid mice. The scAAV9-Des-Luc vector was used as control. Bioluminescence imaging revealed that the full-length Sk-CRM4 resulted in a significant and robust increase in skeletal muscle-specific expression (up to 100-fold), compared to the control vector without Sk-CRM4 , in adult mice with no increased expression in other non-target tissues (Fig. 3 and Supplementary Fig. 4 ). Though the five different Sk-CRM fragments significantly augmented expression in the different skeletal muscle groups and in the heart, the overall effect was more modest (typically 3 to 9-fold) than what could be achieved with the full-length Sk-CRM4 element. This indicates that it is the specific combination of all TFBS clusters within the full-length Sk-CRM4 element that is required to confer high levels of transgene expression in the targeted skeletal muscles and heart. Fig. 3 Screening and validation of Sk-CRM4 fragments. a In vivo bioluminescence imaging at week 2 and week 4 post vector injection and quantification of luciferase expression from the different individual organs of adult CB17/IcrTac/Prkdc scid mice injected intravenously with scAAV9-Des-Luc2 (control, no Sk-CRM ), scAAV9-Sk-CRM4 a -Des-Luc, scAAV9-Sk-CRM4 b -Des-Luc, scAAV9-Sk-CRM c -Des-Luc, scAAV9-Sk-CRM4 d -Des-Luc, and scAAV9-Sk-CRM4 e -Des-Luc vectors at a dose of 1 × 10 10 vg per mouse. The corresponding color scale from 6.70e + 03 (blue) ph/s/cm 2 /sr to 2.70e + 05 (red) ph/s/cm 2 /sr was shown. Photon emission was measured dynamically during 7 min in a supine position. b Ex vivo bioluminescence imaging of individual organs such as the heart and the different muscle groups harvested at 6 weeks post vector injection was represented on a color scale with luciferase intensities ranging from 5.92e + 03 (blue) ph/s/cm 2 /sr to 5.08e + 04 (red) ph/s/cm 2 /sr. The bioluminescence signal was quantified for 5 min. c Luciferase expression from the individual tissues was measured as total flux, expressed in photons/sec/cm 2 /sr. The fold-difference of the total flux was indicated for each Sk-CRM4 fragments relative to that of the control group containing the Des promoter without any Sk-CRM . The total flux data were displayed as mean + s.e.m. ( n = 3) Full size image Comparison of promoter strength with conventional promoters The performance of the Sk-CRM4/Des chimeric promoter was subsequently compared with that of CMV and the synthetic SPc5-12 promoter, commonly used for muscle gene therapy. We also combined the most robust Sk-CRM4 element with the SPc5-12 promoter to assess whether it can further increase its strength, as in the case of the Des promoter. The scAAV9-Sk-CRM4-Des-Luc, scAAV9-Des-Luc, scAAV9-Sk-CRM4-SPc5-12-Luc, scAAV9-SPc5-12-Luc, or scAAV9-CMV-Luc vectors (Fig. 1b–f ) were injected intravenously at a dose of 10 10 vg/mouse in adult CB17/IcrTac/Prkdc scid mice. Bioluminescence analysis in vivo (Fig. 4a ) or ex vivo (Fig. 4b ) on the isolated muscles revealed that the Sk-CRM4/Des combination was the most robust Sk-CRM /promoter combination. In particular, compared to CMV , a significant 25 to 173-fold increase ( t -test; p < 0.01) in transgene expression from the different skeletal muscles could be attained. Moreover, a significant 12 and 18-fold increase ( t -test; p < 0.05) in luciferase expression could be achieved with Sk-CRM4/Des in the diaphragm and heart, respectively (Fig. 4c ). Most importantly, Sk-CRM4/Des also outperformed the SPc5-12 and the Sk-CRM4/SPc5-12 promoters (Fig. 4c ). These results suggested that the Sk-CRM4 element did not only increase expression from the Des promoter but also boosted the performance of the SPc5-12 promoter in skeletal muscle and heart, although to a lesser extent than in the case of the Des promoter. In particular, when comparing the Sk-CRM4/SPc5-12 chimeric promoter with the SPc5-12 promoter, a 15- to 30-fold increase in expression was attained (based on total flux data from different muscles not including diaphragm). This indicates that the Sk-CRM4 element has the potential to augment expression from different muscle-specific promoters, the extent of which varies depending on the intrinsic strength of those promoters. Fig. 4 Comparison of Sk-CRM /promoter combinations with conventional promoters. a In vivo bioluminescence imaging at week 2 and week 4 post vector injection in adult CB17/IcrTac/Prkdc scid mice intravenously injected with the different scAAV9 luciferase vectors containing the different promoters ( CMV, Des, Sk-CRM4/Des, SPc5-12, Sk-CRM4/SPc 5-12 ) at a dose of 1 × 10 10 vg per mouse. A color scale from 6.7e + 03 (blue) ph/s/cm 2 /sr to 2.7e + 05 (red) ph/s/cm 2 /sr was shown. Photon emission was measured dynamically during 7 min. b Ex vivo bioluminescence imaging of individual tissues harvested at 6-week post vector injection was represented on a color scale with luciferase intensities ranging from 3.80e + 03 (blue) ph/s/cm 2 /sr to 2.02e + 04 (red) ph/s/cm 2 /sr. The bioluminescence signal was quantified for 5 min. c Luciferase expression from the individual tissues was measured as total flux, expressed in ph/s/cm 2 /sr. The fold-difference of the total flux of the SkCRM4/Des chimeric promoter was indicated relative to the CMV promoter (without any Sk-CRM) . The luciferase signal were showed as mean + s.e.m. ( n = 3) Full size image Therapeutic validation in a dystrophic mouse model We subsequently validated the performance of the Sk-CRM4/Des chimeric promoter in a preclinical gene therapy setting. We, therefore, generated AAV9 vectors expressing either a truncated codon-usage optimized human micro-dystrophin ( MD1Δ ) (Fig. 1g ) or a human follistatin cDNA ( FST344 ) (Fig. 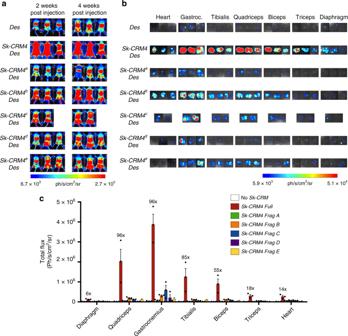Fig. 3 Screening and validation ofSk-CRM4fragments.aIn vivo bioluminescence imaging at week 2 and week 4 post vector injection and quantification of luciferase expression from the different individual organs of adult CB17/IcrTac/Prkdcscidmice injected intravenously with scAAV9-Des-Luc2 (control, noSk-CRM), scAAV9-Sk-CRM4a-Des-Luc, scAAV9-Sk-CRM4b-Des-Luc, scAAV9-Sk-CRMc-Des-Luc, scAAV9-Sk-CRM4d-Des-Luc, and scAAV9-Sk-CRM4e-Des-Luc vectors at a dose of 1 × 1010vg per mouse. The corresponding color scale from 6.70e + 03 (blue) ph/s/cm2/sr to 2.70e + 05 (red) ph/s/cm2/sr was shown. Photon emission was measured dynamically during 7 min in a supine position.bEx vivo bioluminescence imaging of individual organs such as the heart and the different muscle groups harvested at 6 weeks post vector injection was represented on a color scale with luciferase intensities ranging from 5.92e + 03 (blue) ph/s/cm2/sr to 5.08e + 04 (red) ph/s/cm2/sr. The bioluminescence signal was quantified for 5 min.cLuciferase expression from the individual tissues was measured as total flux, expressed in photons/sec/cm2/sr. The fold-difference of the total flux was indicated for eachSk-CRM4fragments relative to that of the control group containing theDespromoter without anySk-CRM. The total flux data were displayed as mean + s.e.m. (n= 3) 1k ). Injection of ssAAV9-Sk-CRM4-Des-MD1Δ by itself or in combination with ssAAV9-Sk-CRM4-Des-FST in SCID/mdx mice resulted in widespread MD1 expression in heart and skeletal muscles (Fig. 5a, b ), consistent with a significant percentage (Fig. 5c ) of dystrophin-positive fibers (DYS + ) in both heart and skeletal muscle compared to untreated control SCID/mdx mice. Similarly, injection of ssAAV9-Sk-CRM4-Des-FST by itself or in combination with AAV9-Sk-CRM4-Des-MD1Δ resulted in significantly higher FST protein levels (Fig. 5d ) expression in skeletal muscle compared to untreated control SCID/mdx mice. These results were consistent with significantly elevated levels of MD1Δ or FST transcripts in transduced skeletal muscle and heart of SCID/mdx mice (Fig. 5e ). Fig. 5 Human MD1 and human FST expression analysis in immunodeficient dystrophic SCID/mdx mice. The ssAAV9-Sk-CRM4-Des-MD1Δ and ssAAV9-Sk-CRM4-Des-FST vectors were injected either alone (indicated as MD1Δ, FST) or in combination (indicated as MD1Δ + FST) in SCID/mdx mice at a dose of 2 × 10 10 vg/mouse. a , b Immunofluorescence staining for laminin (LAM, in green), human dystrophin (DYS, in red) and DAPI nuclear staining (in blue) was performed on sections from heart ( a ) and skeletal muscles ( b ) of treated and untreated control SCID/mdx mice. The scale bars indicate 100 μm. c Quantification of the DYS + fibers detected out of the total number of LAM + fibers in the heart and skeletal muscle tissue sections from treated and untreated control SCID/mdx mice. d Quantification of human FST protein (in pg/50 mg of skeletal muscle tissue) as determined by ELISA. e Human MD1Δ and FST mRNA quantification in the heart and the skeletal muscles (i.e., gastrocnemius, quadriceps) of treated and untreated control SCID/mdx mice, expressed relative to the murine housekeeping gene Gapdh by qRT-PCR. Mice were injected at 4 weeks and euthanized 22 weeks later. The data were represented as mean + s.e.m. ( n = 2–4) Full size image SCID/mdx mice treated with the ssAAV9-Sk-CRM4-Des-MD1Δ and ssAAV9-Sk-CRM4-Des-FST alone or in combination, outperformed the untreated control mice in treadmill test 16 weeks post vector injection (Fig. 6a ). In particular, the performance of dystrophic mice treated with the ssAAV9-Sk-CRM4-Des-MD1Δ or ssAAV9-Sk-CRM4-Des-FST vector increased with 300% ( t -test; p < 0.001) and 250%, respectively, compared to untreated dystrophic mice. Most importantly, the performance of dystrophic mice that received combination gene therapy by co-delivery of both ssAAV9-Sk-CRM4-Des-MD1Δ and ssAAV9-Sk-CRM4-Des-FST showed a robust 356% increase, compared to untreated dystrophic mice (Fig. 6a ). This was consistent with a significant 1.8-fold increase ( t -test; p < 0.05) in absolute tetanic contraction force ex vivo on isolated extensor digitorum longus (EDL) muscle from SCID/mdx mice that received the combination gene therapy, approximating the EDL absolute contraction force in wild-type C57BL/6 mice (191 + 58 mN in MD1Δ/FST-treated SCID/mdx; 105 + 13 mN in untreated SCID/mdx; 232 + 42 mN wild-type C57BL/6). Fig. 6 Phenotypic correction of muscular dystrophy in SCID/mdx mice. a SCID/mdx mice injected with ssAAV9-Sk-CRM4-Des-MD1Δ only, ssAAV9-Sk-CRM4-Des-FST only, and ssAAV9-Sk-CRM4-Des-MD1Δ with ssAAV9-Sk-CRM4-Des-FST combination therapy (2 × 10 10 vg/mouse of each vector) were subjected to a treadmill assay. Physical performance of the 20-week-old SCID/mdx mice treated with the different therapeutic vectors compared to the untreated age-matched control SCID/mdx mice was determined by measuring the distance covered. Results were presented as mean ± standard error of the mean, (% increase in distance covered relative to untreated SCID/mdx was indicated. b – d Improvement of pathophysiological properties in SCID/mdx mice injected with ssAAV9-Sk-CRM4-Des-MD1Δ, ssAAV9-Sk-CRM4-Des-FST, ssAAV9-Sk-CRM4-Des-MD1Δ, and ssAAV9-Sk-CRM4-Des-FST combination therapy. b Hematoxylin and eosin staining of 5 μm thick transverse sections of the tibialis anterior muscle from mice treated with the different therapeutic vectors were compared with those of age-matched control C57BL/6 and SCID/mdx mice treated with PBS. The scale bars indicate 50 μm. c Graphical representation of the % of central nucleation in muscle fibers from treated sections versus the age-matched non-treated sections. Results were presented as mean ± standard error of the mean, *** p < 0.001 and **** p < 0.0001 using Student’s t -test ( n = 4–9). d Muscle fiber cross-sectional area (expressed in pixels) of each of the different groups of SCID/mdx mice treated with the different therapeutic vectors (at a dose of 2 × 10 10 vg/mouse). Untreated SCID/mdx and C57BL/6 mice were used as controls. Results were presented as mean ± standard error of the mean, * p < 0.05; *** p < 0.001, and **** p < 0.0001 using Student’s t -test ( n = 4–5) Full size image We subsequently corroborated the functional correction after gene therapy by histopathological examination of the skeletal muscle. The central localization of the nucleus in the muscle fibers is one of the hallmarks of muscular dystrophy, as opposed to peripheral nuclear localization in normal, non-dystrophic muscle fibers. Hematoxylin and eosin staining of the tibialis anterior muscle revealed a significant reduction ( t -test; p < 0.0001) in centrally nucleated muscle fibers after systemic gene therapy with ssAAV9-Sk-CRM4-Des-MD1Δ and/or ssAAV9-Sk-CRM4-Des-FST compared to non-treated SCID/mdx mice (Fig. 6b, c ). Moreover, the combination therapy based on co-delivery of both ssAAV9-Sk-CRM4-Des-MD1Δ and ssAAV9-Sk-CRM4-Des-FST resulted in an even more pronounced and significant effect ( t -test; p < 0.001) on the nuclear re-localization towards the muscle fiber periphery than by either of the single vector treatments (Fig. 6b, c ). Furthermore, the fiber cross-sectional area also increased after gene therapy with the Sk-CRM4-based vectors. In particular, treatment of SCID/mdx mice with the ssAAV9-Sk-CRM4-Des-MD1Δ vector significantly increased the cross-sectional area 130% ( t -test; p < 0.001) (Fig. 6d ) compared to untreated SCID/mdx mice. The effect was even 250% greater following ssAAV9-Sk-CRM4-Des-FST treatment ( t -test; p < 0.0001), exceeding the fiber cross-sectional area typically observed in wild-type mice (Fig. 6d ). The maximum effect could be attained upon co-delivery of ssAAV9-Sk-CRM4-Des-MD1Δ and/or ssAAV9-Sk-CRM4-Des-FST resulting in a 285% increase in fiber cross-sectional area ( t -test; p < 0.001). In conclusion, the impact of gene therapy on the improvement of the histopathological features characteristic of a dystrophic phenotype was consistent with its effect on overall physical performance and muscle function. Comparative analysis of therapeutic efficiency The performance of the Sk-CRM4/Des chimeric promoter was subsequently compared with other conventional promoters, such as Des and CMV (Fig. 1i, j, l, m ), which are generally used for therapeutic gene expression in skeletal muscles and being used in clinical trials for muscle-directed gene therapy. Comparative functional analysis 16 weeks post-injection (Fig. 7a ) revealed that robust and sustained phenotypic correction could be achieved in SCID/mdx mice co-injected with the ssAAV9-SkCRM4-Des-MD1 (Fig. 1i ) and ssAAV9-SkCRM4-Des-FST (Fig. 1l ) vectors resulting in a normalization of the running distance covered, comparable to that of wild-type mice (Student’s two-tailed t -test; p -value = 0.6245, non-significant). This represent a robust ≈800% improvement in distance traveled compared to the untreated dystrophic SCID/mdx mice ( t -test; p < 0.01). Hence, this is consistent with a bona fide cure of muscular dystrophy in this preclinical model when the next-generation AAV9 vectors that expressed the MD1 and FST genes from the de novo designed SkCRM4-Des promoter. Most importantly, the therapeutic effect was significantly increased ( t -test; p < 0.05) when the SkCRM4/Des promoter was used compared to when the therapeutic MD1 and FST genes were driven from either CMV or Des promoters (Fig. 7a ). Fig. 7 Comparison of Sk-CRM4/Des chimeric promoter with conventional promoters in SCID/mdx. The ssAAV9 vectors encoding MD1 and FST under the control of the Sk-CRM4/Des chimeric promoter, Des , or CMV conventional promoters were co-injected into SCID/mdx mice at a dose of 1 × 10 11 vg/mouse for each vector. a Physical performance of the 16 weeks post-injected SCID/mdx mice treated with the different therapeutic vectors compared to the untreated age-matched control SCID/mdx and wild-type C57BL/10ScSnJ mice were determined by measuring the distance covered. Results were presented as mean ± standard error of the mean ( n = 3–6). The percentages on the top indicate the distance related to untreated SCID/mdx mice. b Human MD1 and FST mRNA quantification in skeletal muscles (i.e., gastrocnemius and quadriceps) of treated SCID/mdx mice, expressed relative to the housekeeping gene Gapdh by qRT-PCR. The Gapdh protein levels were used as loading control for normalization. c Quantification of human FST protein (in pg/50 mg of skeletal muscle tissues) as determined by ELISA. d Western blot analysis of MD1 protein expression in heart, diaphragm and skeletal muscle ( gastrocnemius ) of treated and control SCID/mdx. The protein expression levels of MD1 were detected using a dystrophin-specific (DYS3) antibody. Statistical analysis using t -test * p < 0.05; ** p < 0.01; *** p < 0.001, **** p < 0.0001; mean + s.e.m. ( n = 3–6) Full size image Next, the MD1 and FST mRNA and protein expression levels were determined using qRT-PCR (Fig. 7b ) and ELISA (Fig. 7c ) or western blotting (Fig. 7d ), respectively. The new muscle-specific Sk-CRM4/Des chimeric promoter led to a robust increase in MD1 and FST (Figs. 7b and 8b ) mRNA expression levels compared to when CMV or Des promoters were used, as control. This translated in a significant ( t -test; p < 0.01) increase in MD1 in heart, diaphragm and skeletal muscle ( gastrocnemius) (Fig. 7d ) and FST (Fig. 7c ) protein expression when the Sk-CRM4/Des chimeric promoter was used compared to the CMV or Des promoters. The western blot analysis confirmed that MD1 had the expected molecular weight (136 kD) (Fig. 7d and Supplementary Fig. 6 ). Hence, the increased therapeutic efficacy with the next-generation AAV vectors expressing the MD1 and FST therapeutic genes from the Sk-CRM4/Des chimeric promoter was consistent with the increase in MD1 and FST expression. These results suggested that the use of the Sk-CRM4/Des chimeric promoter provided an effective and sustained therapeutic effect that is significantly more robust compared to conventional promoters typically used for DMD gene therapy. Fig. 8 Comparison of Sk-CRM4/Des chimeric promoter with conventional promoters in mdx mice model. The ssAAV9 vectors encoding MD1 and FST gene under Sk-CRM4/Des chimeric promoter, Des , or CMV were co-injected as a combination therapy into mdx mice at a dose of 1 × 10 11 vg/mouse or 5 × 10 11 vg/mouse. a Treadmill test of the 20-week-old mdx mice (16 weeks post-injection) treated with the different constructs of therapeutic vectors compared to the untreated mdx and wild-type C57BL/10ScSnJ mice. The results were shown as the distance covered. The percentages indicate the distance related to untreated mdx mice. Statistical analysis using t -test * p < 0.05 ( n = 4–5). b Human MD1 and FST mRNA quantification in skeletal muscles, i.e., gastrocnemius and quadriceps of treated mdx mice, expressed relative to the housekeeping gene Gapdh by qRT-PCR. c Quantification of human FST protein as measured using ELISA. Results were presented as mean ± standard error of the mean. Statistical analysis using t -test * p < 0.05, ** p < 0.01 (related to 1 × 10 11 injected group of the same construct), # p < 0.05; mean + s.e.m. ( n = 4–5) Full size image In addition to the SCID/mdx model, the efficacy of the Sk-CRM4/Des constructs for DMD treatment was also validated in an immunocompetent dystrophic mouse model (mdx) and compared with conventional promoters (Fig. 8a–c ). Co-injection of mdx mice with the ssAAV9-SkCRM4-Des-MD1 and ssAAV9-SkCRM4-Des-FST vectors resulted in a significant increase ( t -test; p < 0.05) in therapeutic efficacy based on a treadmill assay, at all vector doses tested, consistent with a significant increase in MD1 or FST mRNA (Fig. 8b ) or protein expression levels (Fig. 8c ). Notably, even at a fivefold lower vector dose (i.e., 10 11 vg) the SkCRM4-Des -containing vectors outperformed the vectors that expressed the MD1 or FST therapeutic transgenes from either the CMV or Des promoters resulting in higher transgene expression levels resulting in a significant increase in overall therapeutic efficacy. Collectively, these results indicate that this new SkCRM4 transcriptional element lowers vector dose requirement. Lastly, we examined the extent of the apoptosis using a TUNEL assay. Analysis of skeletal muscle (tibialis anterior) from mdx mice injected with the different AAV9 vectors expressing MD1 or FST from the SkCRM4-Des, Des or CMV promoters (at 5 × 10 11 vg/mouse for each vector) revealed that there was no significant increase in apoptotic cells compared to untreated control mdx or wild-type control mice (Supplementary Fig. 7a ). Moreover, immunohistochemistry for staining CD4 and CD8-positive T cells in the muscles revealed no significant increase in T-cell infiltration in skeletal muscle from mdx mice injected with the various AAV9 vectors expressing MD1 or FST from the SkCRM4-Des, Des or CMV promoters (Supplementary Fig. 7b ). Hence, this indicates that over-expression of MD1 or FST in the skeletal muscle with the next-generation ssAAV9-SkCRM4-Des-MD1 and ssAAV9-SkCRM4-Des-FST vectors was considered to be relatively safe. In this study, we have identified novel and potent muscle-specific CRMs using an improved genome-wide computational algorithm. In particular, the most potent Sk-CRM4 element resulted in a substantial improvement in transcription (up to 400-fold) when combined with the muscle-specific desmin promoter, one of the most commonly used muscle-specific promoters [35] , [39] , [40] . In addition, a 36-fold increase in cardiac expression could be attained. To our knowledge, this type of computational vector design represents the first of its kind to improve the performance of a gene therapy vector for muscle-directed gene therapy, yielding an unprecedented increase in muscle-specific gene expression. Indeed, our previously identified cardiac-specific CRM failed to increase muscle-specific expression from the synthetic SPc5-12 promoter, in contrast to the present study [41] . Moreover, the muscle-specific Sk-CRM4/Des chimeric promoter outperformed the commonly used CMV promoter, up to 100- to 200-fold in most muscle groups and thus provides an attractive alternative [34] , [42] . In particular, the CMV promoter was employed to drive expression of the lipoprotein lipase (LPL S447X ) gene that constitutes the basis of the first approved AAV-based gene therapy product [6] , [7] . Our current results underscore the potential of these computationally designed CRMs to improve the efficacy of skeletal muscle-directed and cardiac gene therapy of DMD, with broad implications for other muscle disorders. In particular, the combination of the de novo designed Sk-CRM/Des muscle-specific promoter with the use of the AAV9 muscle-tropic serotype resulted in widespread expression of reporter or therapeutic genes (i.e. micro-dystrophin, follistatin) in heart and skeletal muscle following systemic gene delivery in neonatal or adult mice. This was consistent with robust phenotypic correction of the dystrophic phenotype in DMD mice resulting in long-term improvement of the physical performance and restoration of several characteristic dystrophic pathophysiological features, particularly increased muscle fiber size and re-localization of the fiber nuclei from the nuclei towards the periphery. Previous efforts to augment muscle-directed gene expression by promoter optimization and/or AAV capsid engineering typically resulted in more modest and incremental increases in gene expression. Moreover, though muscle-specific promoters are often preferred by virtue of their tissue-specificity, they typically yield much lower expression levels than ubiquitously expressed promoters like CMV [35] that are sometimes prone to transcriptional silencing in vivo [43] . The incorporation of the Sk-CRM4 element upstream of the desmin ( Des ) promoter overcomes this limitation by boosting muscle-specific gene expression levels by several orders of magnitude, based on reporter genes (i.e., luciferase). The generation of synthetic muscle-specific promoters (i.e . , SPc5-12 ) by molecular assembly and selection of muscle-specific TFBS combinations in muscle cell lines in vitro has been proposed as an alternative strategy to boost muscle-specific gene expression [31] , [44] . However, this in vitro selection approach resulted in a relatively modest and incremental six-fold increase in muscle-specific expression relative to the CMV promoter, which is in contrast to the robust 100-fold increased expression attained with the computationally designed Sk-CRM4/Des chimeric promoter relative to CMV . In particular, head-to-head comparative analysis revealed that the Sk-CRM4/Des promoter is 15- to 30-fold more potent than the synthetic SPc5-12 promoter (Fig. 4a–d ). The current computational approach distinguishes itself from this synthetic molecular assembly and in vitro selection method by allowing comprehensive and genome-wide identification of evolutionary conserved TFBS clusters that are associated with highly expressed, muscle-specific genes in human muscle in vivo. Consequently, this translated into a more robust increase in expression after gene therapy in vivo, compared to what could be achieved using synthetic promoters obtained by in vitro assembly and selection [31] , [44] . The different muscle-specific human CRMs were retrieved from their natural in vivo context following a genome-wide screening and contained a molecular signature composed of TFBS clusters (containing TFBS for E2A, CEBP, LRF, MyoD, SREBP, Tal1, PPAR) that are characteristic of highly expressed genes in the muscle. In particular, the Sk-CRM4 and Sk-CRM1 elements are among the most potent muscle-specific CRMs that have several TFBS in common (i.e., E2A, LRF, CEBP , and MyoD ). 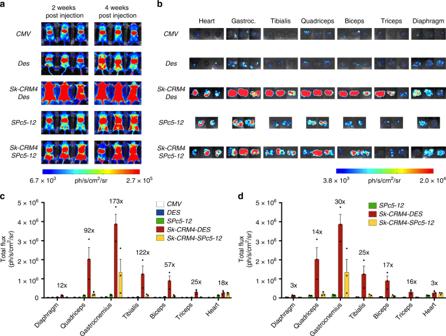Fig. 4 Comparison ofSk-CRM/promoter combinations with conventional promoters.aIn vivo bioluminescence imaging at week 2 and week 4 post vector injection in adult CB17/IcrTac/Prkdcscidmice intravenously injected with the different scAAV9 luciferase vectors containing the different promoters (CMV, Des, Sk-CRM4/Des, SPc5-12, Sk-CRM4/SPc 5-12) at a dose of 1 × 1010vg per mouse. A color scale from 6.7e + 03 (blue) ph/s/cm2/sr to 2.7e + 05 (red) ph/s/cm2/sr was shown. Photon emission was measured dynamically during 7 min.bEx vivo bioluminescence imaging of individual tissues harvested at 6-week post vector injection was represented on a color scale with luciferase intensities ranging from 3.80e + 03 (blue) ph/s/cm2/sr to 2.02e + 04 (red) ph/s/cm2/sr. The bioluminescence signal was quantified for 5 min.cLuciferase expression from the individual tissues was measured as total flux, expressed in ph/s/cm2/sr. The fold-difference of the total flux of theSkCRM4/Deschimeric promoter was indicated relative to theCMVpromoter (without anySk-CRM). The luciferase signal were showed as mean + s.e.m. (n= 3) They were derived from quintessential human muscle-specific genes MYLPF and APTP2A1 that encode for the myosin light chain and the sarcoplasmic/endoplasmic CA 2+ ATPase (SERCA), respectively. Since MYLPF and APTP2A1 are typically highly expressed in fast twitch muscle, this may possibly account for the higher activity of Sk-CRM4 and Sk-CRM1 in the fast twitch skeletal muscles, whereas their activity was lower in low twitch muscle, like diaphragm. Nevertheless, the reduced gene transfer in the diaphragm compared to that in other muscles may also have contributed to the reduced gene expression (Supplementary Fig. 2 ). The increased protein expression from the CRM -driven constructs correlated strongly with increased transcriptional activity. This was consistent with the increased binding of CEBP and SRF on the MYLPF promoter regions encompassing the respective TFBS that were mapped within the Sk-CRM4 element. The main advantage of this novel computational approach used to identify the tissue-specific CRMs is that it takes into account the actual context-dependent TFBS interactions from a broad genome-wide perspective in vivo, instead of just relying on the over-representation of a single TFBS in a given tissue-specific CRM . Consequently, this computational analysis is more comprehensive and allows for the identification of TFBS elements that tend to cluster together in CRMs of genes that are highly expressed in the skeletal muscle and the heart (Table 1 ), based on a differential distance matrix-multidimensional scaling (DDM-MDS) [45] . DDM-MDS is a count-based method that evaluates the statistical significance of the observed versus expected numbers of TFBSs in the sets of promoters. The main difference with methods that only consider over-representation is that a data structure is used that allows simultaneous evaluation of the degree of association between TFBSs for different TFs. The DDM-MDS method [45] produces more relevant and/or reproducible results compared to other methods such as LogicMotif [46] , POCO [47] , and CRÈME [48] . Another advantage of this DDM-MDS approach is does not need to rely on a comprehensive database containing all muscle-specific genes, but merely a gene set corresponding to the most highly expressed genes, The analysis is most robust if we restrict ourselves to a selection of these most highly expressed muscle-specific genes rather than a comprehensive list of all muscle-specific genes (see Supplementary Method). In the current study, the analysis was based on 29 promoters which falls in a similar range as our recent studies, that are based on 43 or 59 to identify cardiac-specific or liver-specific CRMs, respectively [41] , [49] , [50] . Our computational approach takes into account cross-species evolutionary conservation of the selected Sk-CRM elements (Supplementary Fig. 1 ). Cross-species comparison significantly improves genome-wide prediction of CRMs [51] , [52] . This justifies prioritizing CRMs based on evolutionary conservation. Consequently, such evolutionary conserved CRMs are likely to exhibit the same properties across distinct species with respect to tissue-specificity and expression levels. This is important for gene therapy as tissue-specificity and expression levels based on a given CRM may then likely be conserved in preclinical models and human subjects. This potentially improves the prospects for clinical translation. Indeed, if a sequence is conserved and is associated with highly expressed genes in a given species, it will likely be associated with high expression in other species as well. Nevertheless, evolutionary conservation in as of itself does not necessarily imply that the CRMs are evolutionarily optimized and selected for to maximize expression. Open chromatin structures, as defined in the ENCODE database [53] were considered in the current computational analysis, which distinguishes the current approach from our previous strategies used to maximize tissue-specific gene expression after gene therapy [41] , [49] , [50] . We, therefore, considered chromatin contextual features better describing features like DNA accessibility, nucleosome occupancy, or the presence of specific histone post-translational modifications associated with transcription regulation. In practice, candidate Sk-CRMs were mapped against the human hg19 genome using the blat tool at the UCSC genome browser ( https://genome.ucsc.edu ). Next, the mapped regions were visualized along the ENCODE Regulation supertrack containing information relevant to regulation of transcription from the ENCODE project. 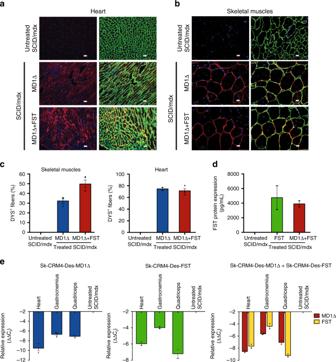Fig. 5 Human MD1 and human FST expression analysis in immunodeficient dystrophic SCID/mdx mice. The ssAAV9-Sk-CRM4-Des-MD1Δ and ssAAV9-Sk-CRM4-Des-FST vectors were injected either alone (indicated as MD1Δ, FST) or in combination (indicated as MD1Δ + FST) in SCID/mdx mice at a dose of 2 × 1010vg/mouse.a,bImmunofluorescence staining for laminin (LAM, in green), human dystrophin (DYS, in red) and DAPI nuclear staining (in blue) was performed on sections from heart (a) and skeletal muscles (b) of treated and untreated control SCID/mdx mice. The scale bars indicate 100 μm.cQuantification of the DYS+fibers detected out of the total number of LAM+fibers in the heart and skeletal muscle tissue sections from treated and untreated control SCID/mdx mice.dQuantification of human FST protein (in pg/50 mg of skeletal muscle tissue) as determined by ELISA.eHumanMD1ΔandFSTmRNA quantification in the heart and the skeletal muscles (i.e., gastrocnemius, quadriceps) of treated and untreated control SCID/mdx mice, expressed relative to the murine housekeeping gene Gapdh by qRT-PCR. Mice were injected at 4 weeks and euthanized 22 weeks later. The data were represented as mean + s.e.m. (n= 2–4) The layered H3K4Me1 and layered H3K27Ac marks are epigenetic signatures often found near regulatory elements, while the DNase I hypersensitivity tracks indicate where chromatin is hypersensitive to cutting by DNase I and are associated with both regulatory regions and promoters. The open chromatin structure is used as a filter in the selection of candidate CRMs because this indicates that, at least in some conditions, a particular genomic region is accessible to TFs. In contrast, some chromatin features may reduce the accessibility of the DNA and therefore impede expression, despite the presence of other favorable features. Moreover, chromatin effects are known to influence expression from AAV vectors as AAV adopts a chromatin-like configuration [54] , [55] , [56] . Enhancers typically activate gene expression when they are located at far greater distances from the transcriptional start site ( TSS ). However, such distal enhancers may increase the risk of insertional oncogenesis following vector integration in the target cell genome [57] , [58] . Hence, we strategically focused on selecting CRMs that are located within the proximal promoter (i.e., < 2.5 kb from TSS ) to diminish the risk of insertional oncogenesis when used in the context of gene therapy. We have previously demonstrated that CRMs that have been identified with the DDM-MDS method and that are located within a 2 kb region from the TSS (i.e., HS-CRM8 [49] , [50] ), do not significantly increase the risk of insertional oncogenesis, in normal or highly sensitive tumor-prone mouse models, even when vectors are employed that integrate at high efficiencies in the target cell genome [59] . The overall efficiency of this next-generation AAV-based muscle-directed gene therapy compares favorably to the state of the art vectors as higher expression levels could be attained leading to an increased therapeutic efficacy. Previous studies were based on intramuscular AAV injections, which did not allow body-wide expression of the therapeutic micro-dystrophin and consequently resulted in a more modest correction of the dystrophic phenotype [30] , [60] . Moreover, substantial correction of the dystrophic phenotype could be achieved in a physical endurance test (i.e., treadmill assay) either using a single or a combination of therapeutic genes (i.e., MD1 or FST ). The overall impact of the Sk-CRM4 element on gene expression may vary depending on the transgene. Indeed, though the Sk-CRM4 element led to a significant increase in both MD1 and FST transcription, the highest relative- increase in mRNA levels was apparent when luciferase was used. Moreover, the significant increase in MD1 and FST protein levels was not directly proportionate to the increased transcription. This suggests that additional, potentially unknown, post-transcriptional or translational bottlenecks may influence gene therapy efficacy. Though over-expressing a potential therapeutic gene might lead to imbalanced protein synthesis followed by muscle fiber death, lack of apoptosis or T-cell infiltration further supports the safety of the current vector designs and allowed for the use of lower vector doses to attain an increased therapeutic effect compared to more conventional vector designs. Other studies that were based on systemic intravenous injection of AAV vectors encoding therapeutic genes typically required higher vector doses than the therapeutic doses used in the present study [16] , [17] and/or requiring the use of vascular endothelial growth factor (VEGF 164 ), raising additional safety concerns. Lower vector doses may minimize the risk of potential AAV-specific T-cell immune response in human trials and may ease manufacturing constraints. The first gene therapy trials for DMD had been initiated based on intramuscular delivery of an AAV2.5 variant encoding mini-dystrophin [20] . Overall, dystrophin-expression in patient’s biopsies was either absent or limited. Similarly, the use of oligonucleotide-based exon-skipping approaches failed to demonstrate any long-term effects [25] , [61] . The next-generation vector design described in the present study may potentially overcome some of these bottlenecks and pave the way towards clinical applications to treat DMD and other muscle disorders. Identification of Sk-CRM We designed a computational approach (Fig. 1a ) (Supplementary Methods) to specifically identify robust skeletal muscle CRMs ( Sk-CRMs) . This approach consisted of five steps: (1) muscle-specific genes were identified that are highly and lowly expressed based on statistical analysis of micro-array expression data of normal human tissues; [62] , [63] (2) publicly available databases were used to extract the corresponding promoter sequences (NCBI36/hg18 genome assembly) (3) a differential distance matrix (DDM)-multidimensional scaling (MDS) approach [45] was used to identify the regulatory modules and the TFBS they contain (4) the genomic context of the highly expressed genes was then screened for evolutionary conserved clusters of TFBS (i.e., CRMs ). A detailed description of these four successive steps for identification of tissue-specific CRM was described, that led to the identification of robust liver-specific or cardiac-specific CRMs [41] , [49] , [50] . However, in the present study we further refined this computational analysis by adding an extra step that also takes into consideration biochemical features associated with transcription regulation and/or open chromatin structures, as defined in the ENCODE database (Supplementary Methods) [53] . Six different Sk-CRMs were selected based on this computational analysis (Table 1 ). Generation of Sk-CRMs AAV constructs The CRMs were synthesized by conventional oligonucleotide synthesis (Geneart, Thermo Fisher Scientific, Carlsbad, California, USA) and were flanked with MluI and Acc65I restriction sites at the 5ʹ and 3ʹ’ ends, respectively. After synthesis, the Sk-CRMs were cloned upstream of the desmin ( Des ) promoter (983 bp) (Invivogen, France) in a self-complementary adeno-associated viral ( scAAV ) vector [64] (kindly provided by Dr. Srivastava, University of Florida College of Medicine, USA). 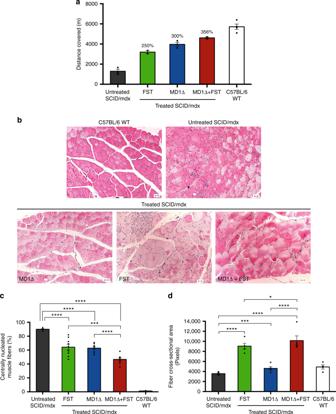Fig. 6 Phenotypic correction of muscular dystrophy in SCID/mdx mice.aSCID/mdx mice injected with ssAAV9-Sk-CRM4-Des-MD1Δ only, ssAAV9-Sk-CRM4-Des-FST only, and ssAAV9-Sk-CRM4-Des-MD1Δ with ssAAV9-Sk-CRM4-Des-FST combination therapy (2 × 1010vg/mouse of each vector) were subjected to a treadmill assay. Physical performance of the 20-week-old SCID/mdx mice treated with the different therapeutic vectors compared to the untreated age-matched control SCID/mdx mice was determined by measuring the distance covered. Results were presented as mean ± standard error of the mean, (% increase in distance covered relative to untreated SCID/mdx was indicated.b–dImprovement of pathophysiological properties in SCID/mdx mice injected with ssAAV9-Sk-CRM4-Des-MD1Δ, ssAAV9-Sk-CRM4-Des-FST, ssAAV9-Sk-CRM4-Des-MD1Δ, and ssAAV9-Sk-CRM4-Des-FST combination therapy.bHematoxylin and eosin staining of 5 μm thick transverse sections of the tibialis anterior muscle from mice treated with the different therapeutic vectors were compared with those of age-matched control C57BL/6 and SCID/mdx mice treated with PBS. The scale bars indicate 50 μm.cGraphical representation of the % of central nucleation in muscle fibers from treated sections versus the age-matched non-treated sections. Results were presented as mean ± standard error of the mean, ***p< 0.001 and ****p< 0.0001 using Student’st-test (n= 4–9).dMuscle fiber cross-sectional area (expressed in pixels) of each of the different groups of SCID/mdx mice treated with the different therapeutic vectors (at a dose of 2 × 1010vg/mouse). Untreated SCID/mdx and C57BL/6 mice were used as controls. Results were presented as mean ± standard error of the mean, *p< 0.05; ***p< 0.001, and ****p< 0.0001 using Student’st-test (n= 4–5) This vector encoded for the firefly luciferase ( Luc ) reporter gene and also contained the Minute Virus of Mouse ( MVM ) intron and a simian virus 40 (SV40) polyadenylation site ( pA ). The corresponding scAAV constructs that contained these Sk-CRM elements were designated as pscAAV-Sk-CRM-Des-Luc (Fig. 1c ). An AAV vector without the Sk-CRM was used as control (designated as pscAAV-Des-Luc ) (Fig. 1b ). For comparison, the most robust Sk-CRM4 (Supplementary Table 1 ) was cloned in combination with a synthetic promoter (SPc5-12) [31] , known for expression in the skeletal muscle and heart, within the scAAV vector backbone to drive the luciferase reporter (designated as pscAAV-Sk-CRM4-SPc5-12-Luc) (Fig. 1f ). The corresponding control AAV vector without the Sk-CRM4 was also generated (designated as pscAAV-SPc5-12-Luc ) (Fig. 1e ). Additionally, the cytomegalovirus promoter ( CMV ) [17] , often used as gold standard to achieve high expression in the muscle, was cloned into the scAAV backbone encoding luciferase for comparison (designated as pAAV-CMV-Luc-SV40pA) (Fig. 1d ). Next, five different sub-fragments of Sk-CRM4 were synthesized by conventional oligonucleotide synthesis and were cloned upstream of the desmin promoter in the same scAAV backbone encoding luciferase. The constructs generated were designated as pssAAV- Sk-CRM (a-e) - Des-Luc . In order to validate these CRMs for gene therapy of DMD, we cloned human micro-dystrophin 1 ( MD1 ) [30] or an alternative truncated version ( MD1Δ ) containing additional deletions of the spectrin-like repeats (Supplementary Fig. 5 ) and human follistatin ( FST344 ) [34] cDNA into a single-stranded AAV (ssAAV) vector driven from the Sk-CRM4/Des chimeric promoter. The MD1 cDNA was flanked by MluI and XhoI restriction sites at the 5ʹ and 3ʹ ends while the FST cDNA was flanked by MluI and SalI restriction sites at the 5ʹ and 3ʹ, respectively, and were synthesized by conventional oligonucleotide synthesis. The Sk-CRM4/Des was cloned upstream of the MVM intron to drive the expression of the MD1 gene or FST gene in the context of a single-stranded adeno-associated viral vector (ssAAV) backbone that also contained a 49 bp synthetic polyadenylation site [65] . The constructs were designated as pssAAV-Sk-CRM4-Des-MD1 (Fig. 1h ) and pssAAV-Sk-CRM4-Des-FST (Fig. 1k ), respectively. In this vector, the FST cDNA was linked to a Luc reporter gene via a 2A polypeptide-encoding fragment. Cloning details are available upon request. AAV vector production and purification AAV vectors were prepared as described in the Supplementary Methods [36] . Genome-containing vectors and empty AAV capsid particles were purified by cesium chloride gradient. The vector titer (in vector genomes or vg/ml) for all vectors was determined by quantitative (q)PCR (Supplementary Methods). Typically, vector titers achieved for all vectors were in the range of 5 × 10 11 –2 × 10 12 vg/ml. Mice This study was carried out in CB17/IcrTac/Prkdc scid mice (Taconic, Denmark), C57BL/6 mice (Janvier Labs, France) or SCID/mdx mice (kindly provided by Dr. Y. Torrente and Mrs. M. Meregalli, University of Milan, Italy). The dystrophic mdx and CB57BL/10ScSnj mice models were purchased from Jackson Laboratory, USA. All animal procedures were carried out at the Vrije Universiteit Brussel and the University of Leuven (Belgium) and were approved by the respective Institutional Animal Ethics Committees (i.e., KU Leuven & VUB Ethische Commissie Dieren—ECD). Mice were housed under specific pathogen-free (SPF)-like conditions; food and water were provided ad libitum. For each cohorts of various experiments, mice were randomly selected from a group of mice of same age and similar weight to standardize control and experimental groups as much as possible. Mice and samples were coded based on the ear tag number. The ear tag number was decoded after conducting the experiment. The designated investigator injecting the vectors was blinded to the experimental outcome. The investigators were blinded to the precise nature of the CRMs or vectors. In vivo bioluminescence analysis For the in vivo screening of the AAV vectors containing the different Sk-CRMs and the Luc reporter gene, 2-days old CB17/IcrTac/Prkdc scid mice were intravenously injected into the retro-orbital vein with 50 μl of purified AAV9 vectors (5 × 10 9 vg/mouse). The experimental mice were subjected to bioluminescence imaging analysis at 5 and 6 weeks post-injection using an in vivo optical imaging system (PhotonImager, Biospace Lab, Paris, France). Alternatively, AAV9 vectors were injected intravenously into the tail vein into adult 6-weeks-old CB17/IcrTac/Prkdc scid adult mice at a dose of 1 × 10 10 vg per mouse and analyzed by bioluminescence imaging 2 and 4 weeks post-injection. Before imaging, mice were intravenously administered with a d -luciferin substrate (30 mg/ml) at a dose of 150 mg/kg of body weight. Quantitative image analysis of individual organs was performed at 7 weeks post vector injection for the mice that were injected as neonates and at 6 weeks post vector injection for the injected adult cohorts. In this case, mice were euthanized by cervical dislocation within 1-minute post d -luciferin administration. In vivo bioluminescence was expressed in photons (ph) s -1 cm -2 steradian (sr) -1 and displayed as a pseudo-color overlay onto a gray scale animal image using a rainbow color scale. All images were scaled to the same maximum and minimum, as represented in the color bar. Transduction efficiency, biodistribution, and mRNA levels Transduction efficiency and biodistribution was evaluated by quantifying Luc transgene copy numbers in the different organs and tissues, as described in Supplementary Methods. The qPCR results were expressed as mean AAV copy number/100 ng of genomic DNA. To quantify Luc mRNA levels in different tissues real-time qPCR analysis was performed using Luc -specific primers (amplicon 206 bp) (Supplementary Methods). All results were normalized to mRNA levels of the endogenous murine glyceraldehyde-3-phosphate dehydrogenase ( Gapdh ) gene (amplicon 82 bp). Chromatin immunoprecipitation assay (ChIP assay) To verify the biding of selected TF on the cognate TFBS , ChIP assays were performed (Supplementary Methods) [67] . Genomic DNA regions of interest were isolated using 4 μg of SRF-specific antibody (sc-335; Santa Cruz Biotechnology, Santa Cruz, CA, USA) or a CEBP-specific antibody (sc-150; Santa Cruz Biotechnology, Santa Cruz, CA, USA). qPCR reactions were carried out in triplicate on specific genomic regions using SYBR Green Supermix (Bio-Rad, USA). 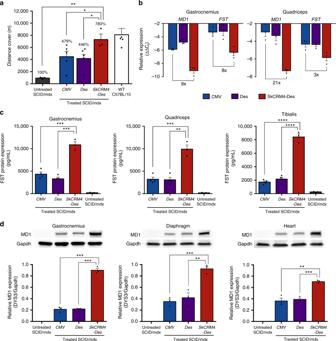Fig. 7 Comparison ofSk-CRM4/Deschimeric promoter with conventional promoters in SCID/mdx. The ssAAV9 vectors encodingMD1andFSTunder the control of theSk-CRM4/Deschimeric promoter,Des, orCMVconventional promoters were co-injected into SCID/mdx mice at a dose of 1 × 1011vg/mouse for each vector.aPhysical performance of the 16 weeks post-injected SCID/mdx mice treated with the different therapeutic vectors compared to the untreated age-matched control SCID/mdx and wild-type C57BL/10ScSnJ mice were determined by measuring the distance covered. Results were presented as mean ± standard error of the mean (n= 3–6). The percentages on the top indicate the distance related to untreated SCID/mdx mice.bHumanMD1andFSTmRNA quantification in skeletal muscles (i.e., gastrocnemius and quadriceps) of treated SCID/mdx mice, expressed relative to the housekeeping gene Gapdh by qRT-PCR. The Gapdh protein levels were used as loading control for normalization.cQuantification of human FST protein (in pg/50 mg of skeletal muscle tissues) as determined by ELISA.dWestern blot analysis of MD1 protein expression in heart, diaphragm and skeletal muscle (gastrocnemius) of treated and control SCID/mdx. The protein expression levels of MD1 were detected using a dystrophin-specific (DYS3) antibody. Statistical analysis usingt-test *p< 0.05; **p< 0.01; ***p< 0.001, ****p< 0.0001; mean + s.e.m. (n= 3–6) 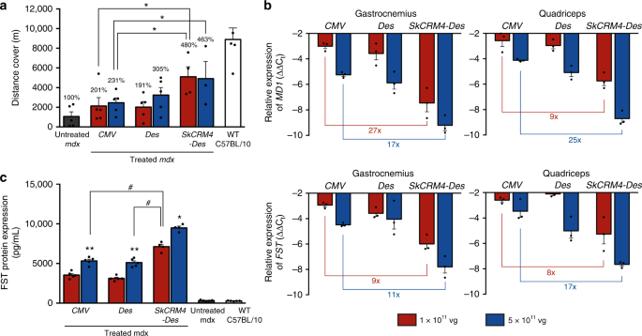Fig. 8 Comparison ofSk-CRM4/Deschimeric promoter with conventional promoters in mdx mice model. The ssAAV9 vectors encodingMD1andFSTgene underSk-CRM4/Deschimeric promoter,Des, orCMVwere co-injected as a combination therapy into mdx mice at a dose of 1 × 1011vg/mouse or 5 × 1011vg/mouse.aTreadmill test of the 20-week-old mdx mice (16 weeks post-injection) treated with the different constructs of therapeutic vectors compared to the untreated mdx and wild-type C57BL/10ScSnJ mice. The results were shown as the distance covered. The percentages indicate the distance related to untreated mdx mice. Statistical analysis usingt-test *p< 0.05 (n= 4–5).bHumanMD1andFSTmRNA quantification in skeletal muscles, i.e., gastrocnemius and quadriceps of treated mdx mice, expressed relative to the housekeeping geneGapdhby qRT-PCR.cQuantification of human FST protein as measured using ELISA. Results were presented as mean ± standard error of the mean. Statistical analysis usingt-test *p< 0.05, **p< 0.01 (related to 1 × 1011injected group of the same construct), #p< 0.05; mean + s.e.m. (n= 4–5) The resulting signals were normalized for primer efficiency by carrying out qPCR for each primer pair using the genomic input DNA with Sk-CRM4- specific forward and reverse primers. Negative control primers were purchased from Active Motif (Carlsbad, CA, USA) (#71012) and are specific for non-transcribed gene sequences on chromosome 17. Analysis of therapeutic efficacy in vivo Four-weeks-old SCID/mdx or mdx mice were injected intravenously into the tail vein with the indicated doses of the ssAAV9-Sk-CRM4-Des-MD1 (or ssAAV9-Sk-CRM4-Des-DM1Δ) and/or ssAAV9-Sk-CRM4-Des-FST therapeutic vector. Control mice were injected with phosphate buffered saline (PBS). Sixteen weeks post-injection, the treated and control SCID/mdx or mdx mice and wild-type age-matched C57BL/6 or C57BL/10ScSnJ mice were subjected to a treadmill test (Exer-3/6 open treadmill, Columbus Instruments, USA) to determine correction of the dystrophic phenotype. The inclination of the belt was adjusted to 10° uphill before performing the test. The initial speed was set at 10 m min -1 and thereafter the speed was increased by 1 m min -1 every minute. The test was terminated at a point when the mice sat for ≥ 5 s on the pulse grill. At that point the distance covered by the mice was recorded and the total distance covered by the mice during the course of the test was calculated by using the formula, according to the manufacturer’s instructions: distance (in m) = ( N + n )/2)*( N − n + 1 ) where N is the speed (in m min -1 ) at the point of termination of the test and n is the speed (in m min -1 ) at the start point of the test. In vitro analysis of muscle contractile properties Mice injected with the ssAAV9-Sk-CRM4-Des-MD1Δ and ssAAV9-Sk-CRM4-Des-FST vectors (2 × 10 10 vg per mouse) were euthanized 18 weeks post vector administration and the extensor digitorum longus muscle was isolated from each mouse to perform the force test. Age-matched C57BL/6 mice and untreated SCID/mdx mice were used as controls. Functional analysis was performed using an Aurora 1200 A in vitro muscle test system, as previously reported [67] . Briefly, freshly isolated muscles were electrically stimulated in a temperature-controlled (30° C) chamber, filled with Krebs-Ringer bicarbonate buffer solution containing 10 mM glucose and continuously gassed with 99% O 2 . The electrical stimulation was performed by means of a couple of platinum electrodes, located 4 mm from each side of the muscle. Tetanic force was evoked by stimulation with a train of 0.2 ms pulses (150 Hz pulses for 0.5 s). Histological analysis Mice injected with the ssAAV9-Sk-CRM4-Des-MD1Δ and ssAAV9-Sk-CRM4-Des-FST vectors (2 × 10 10 vg per mouse) were euthanized 18 weeks post vector injection and the tibialis anterior muscles were harvested for hematoxylin and eosin staining and (Supplementary Methods). For immunofluorescence staining, the heart and the tibialis anterior muscles were subjected to cryofixation and stained for mouse laminin and human dystrophin using specific antibodies and the appropriate fluorescein-isothyocyanate (FITC) or tetramethylrhodamineisothiocyanate-conjugated (TRITC) anti-mouse or anti-rabbit (1:500, Life Technologies, Carlsbad, CA, USA) (Supplementary Methods). Nuclear staining was performed using 4’,6-diamidino-2-phenylindole (DAPI; Hoechst nucleic acid stain, Life technologies, USA) (1:1000 dilution) for 1 h at room temperature. For assessment of the immune response, infiltration of CD4 + and CD8 + T-cells was analyzed. CD4 and CD8-specific antibodies (1:500; Cell signaling, USA) were used as primary antibody to detect mouse T cells. After washing, the samples were subjected to HRP-conjugated secondary antibody (1:2000; Abcam, UK). Substrate was added (3,3’-diaminobenzidine tetrahydrochloride) (DAB kit, Cell signaling, USA) and tissue sections were counterstained using hematoxylin. Spleen sections were used as control. Cellular apoptosis was assessed in situ based on a TUNEL assay. Modified dUTPs were, therefore, incorporated by the enzyme terminal deoxynucleotidyl transferase (TdT) at the 3’-OH ends of fragmented DNA using Click-iT® TUNEL Alexa Fluor647® Imaging Assay (Life Technologies, Carlsbad, CA, USA), according to the manufacturing protocol. Tissue samples were then analyzed under a fluorescent microscope (Nikon Eclipse 80i) and images were processed by NIS Elements 4.30.02 software. FST enzyme-linked immunosorbent assay Human FST was quantified from the muscles of SCID/mdx mice by an enzyme-linked immunosorbent assay (ELISA) with a human FST-specific immunoassay kit (Quantikine; R&D Systems, Minneapolis, USA), according to the manufacturer’s protocol. Briefly, total soluble protein was extracted from 50 mg gastrocnemius, quadriceps, and/or tibialis anterior muscle with CelLytic MT Mammalian Tissue Lysis reagent (Sigma, St. Louis, Missouri, USA). A total of 100 μl of lysate was loaded per well, and muscle FST concentrations were determined against a standard curve made with recombinant human FST provided by the manufacturer. Western blotting Proteins were extracted from skeletal muscles, diaphragm, or heart by solubilization in lysis buffer (50 mM Tris, 5 mM EDTA, 5% sodium dodecyl sulfate, 5% glycerol) supplied with 1x protease inhibitor cocktails (Thermo Fisher Scientific, USA). The total protein concentrations were determined using RC DC™ Protein Assay (Bio-Rad, USA), per manufacturer’s protocol. Then 50–100 microgram of proteins were mixed with sample buffer (Bio-Rad, USA) and loaded into 4–15% TGX gels (Bio-rad, USA) for sodium dodecyl sulfate-polyacrylamide gel electrophoresis. The proteins were transferred to 0.45 μm polyvinylidene fluoride membranes (Invitrogen, USA) using Towbin buffer (Bio-rad, USA). Membranes were blocked with 3% blotting-grade blocker (Bio-rad, USA) for 1 h at room temperature following by incubation with 1:100 mouse anti-human dystrophin antibody (NCL-DYS3; Novocatsra, UK) or 1:1000 rabbit anti-GAPDH antibody (#2118; Cell Signaling Technology, Netherland) in 3% Blotting-grade blocker. After washing three times with 1x TBS-T buffer, the secondary antibodies compatible with primary antibody, e.g., horseradish peroxidase (HRP)–conjugated 1:2000 goat anti-mouse (#7076; Cell Signaling Technology, Netherland) and 1:10,000 goat anti-rabbit IgG (#7074; Cell Signaling Technology, Netherland) were incubated with the membranes for 1 h at room temperature. Afterward, membranes were washed three times for 5 min each with TBS-T buffer. The chemiluminescent signal was developed using the SuperSignal West Pico PLUS substrate (Thermo Fisher Scientific, USA). The sizes of protein were estimated using MagicMarker XP Protein Standard (LC5602; Invitrogen, USA) (Supplementary Fig. 6 ). The signals were quantified under Image-J software. Statistics Data were analyzed using Microsoft Excel Statistics package or Prism Graphpad. Values shown in the figures are the mean + s.e.m. Specific values were obtained by comparison using t -test or one-way ANOVA. Samples were tested ( n = 3–5, twice) and representative results are shown. Reporting summary Further information on experimental design is available in the Nature Research Reporting Summary linked to this article.